Untethered micro-robotic coding of three-dimensional material composition Complex functional materials with three-dimensional micro- or nano-scale dynamic compositional features are prevalent in nature. However, the generation of three-dimensional functional materials composed of both soft and rigid microstructures, each programmed by shape and composition, is still an unsolved challenge. Here we describe a method to code complex materials in three-dimensions with tunable structural, morphological and chemical features using an untethered magnetic micro-robot remotely controlled by magnetic fields. This strategy allows the micro-robot to be introduced to arbitrary microfluidic environments for remote two- and three-dimensional manipulation. We demonstrate the coding of soft hydrogels, rigid copper bars, polystyrene beads and silicon chiplets into three-dimensional heterogeneous structures. We also use coded microstructures for bottom-up tissue engineering by generating cell-encapsulating constructs. Three-dimensional (3D) functional micro-materials have gained significant attention due to their broad applications [1] , [2] , [3] , [4] , [5] . Of particular interest is bioprinting, which has been used to fabricate complex functional materials such as a 3D printed microbattery [5] , bionic ear [6] and tissue-like structures [2] . These 3D complex architectures lack reconfigurability and reversibility features, as the link between the material and the device is not dynamic and the material state is fixed subsequent to material ejection or polymerization due to the nature of bioprinting [2] , [5] , [6] , [7] , [8] . Errors in coding intricacy of 3D functional materials, such as the misplacement of an ejected droplet or clogging can cause bioprinting to fail owing to the irreversibility of the process. Moreover, simultaneous coding of rigid and soft micro-components into 3D functional materials has presented a significant challenge. On the other hand, more traditional methods, for example, by photolithographically defined processes, have excelled at two-dimensional (2D) coding of a variety of materials. Nevertheless, both the inclusion of arbitrary materials and the out-of-plane coding of material composition remain a challenge. To overcome these challenges, the fabrication of soft tissue-like constructs has been performed using a selection of prefabricated 2D or 3D functional micro-parts [9] via microfluidics [10] , [11] , acoustics [12] , magnetics [13] , [14] , multilayer crosslinking [8] and capillary attraction [15] . Microfluidic assembly [10] , [11] and multilayer crosslinking [8] methods perform high-precision assembly without reconfigurability of micro-components, while acoustic [12] and magnetic [13] , [14] methods are capable of disassembling and reassembling microparts with lower precision. However, few of these methods have shown the manipulation of building blocks with a high precision at tens of microns [10] , [11] , [16] , [17] , [18] and none of them has yet presented the coding of a group of soft and rigid materials together with reconfigurability. In this paper, we present a versatile method to code 2D and 3D complex functional materials using untethered magnetic micro-robots. Spatiotemporal control of crawling micro-robots allows for the creation of 3D complex materials composed of functional micro-components with dynamic coding and reconfigurability. This approach offers high precision in 2D and 3D, as well as the capability to code a combination of soft and rigid materials together. The coding resolution is tens of micrometers and can be adjusted with the size of the micro-robot and the resolution of real-time imaging. Advantages of robotic coding include increased capability in the creation of heterogeneous structures made from a variety of materials, on-demand assembly and reconfigurability when flexibility is needed, or dynamic manipulation capability to create structures in a time-dependent process. Here, we spatiotemporally coded a heterogeneous group of objects including rigid copper bars, polystyrene beads, silicon chiplets, polydimethylsiloxane (PDMS) blocks and cell-encapsulating hydrogels in a fluid environment suitable for cell growth and culture. Microgel and micro-robot fabrication and actuation To fabricate hydrogels at scales of a few hundred microns to a millimeter, photocrosslinkable hydrogel precursor solution was first placed between spacers on a glass slide ( Fig. 1a ). Hydrogel geometries were defined by the dimension of the grids in the customized mask and the spacer thickness ( Fig. 1b ). Hydrogels of different shapes were fabricated by exposing the gel precursor solution to UV light and were stored in phosphate-buffered saline (PBS) (see Methods ). To code building units into 2D and 3D complex materials, an untethered magnetic robot with dimensions of 750 μm × 750 μm × 225 μm was placed on the bottom surface of an assembly chamber ( Fig. 1d ). The magnetic robot is composed of neodymium–iron–boron (NdFeB) particles encapsulated in a polyurethane binder and is actuated by a system of eight electromagnets surrounding the workspace. Hydrogels were pushed by micro-robots controlled by algorithms, which dynamically regulates the magnetic field in response to high-level user inputs [19] . Magnetic forces are applied directly to the micro-robot to induce translation, and small oscillatory magnetic torques are applied to break surface friction, which often dominates such microscale contacts [19] . Serial robotic pick-and-place assembly and coding of hydrogels in 2D or 3D was followed by a secondary crosslinking to stabilize the resulting material. The transportation of several hydrogel sizes and shapes across the polyester substrate is quantified in Fig. 1e and Supplementary Fig. 1 . 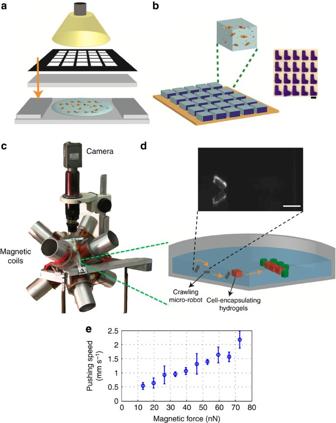Figure 1: Fabrication and micro-robotic coding of cell-encapsulating hydrogels. (a) Cell-encapsulating hydrogel fabrication via ultraviolet (UV) photocrosslinking. (b) Fabricated hydrogels and micrograph of L-shaped hydrogels. Scale bar, 1 mm. (c) Magnetic coil system used to drive magnetic micro-robots remotely. All system components are shown with the coils in the operational position. Two coils hinge open to allow for access to the workspace. (d) Motion of untethered magnetic micro-robot and coding of building units, for example soft hydrogels or rigid micro-components. Scale bar, 1 mm. (e) The pushing speed of a microgel (gel style F inSupplementary Table 1) by a 750 μm × 750 μm × 225 μm micro-robot moving on a planar glass surface in phosphate-buffered saline solution. Error bars represent standard error of the mean. The micro-robot motion was guided by a magnetic force of varying magnitude. Average speed is shown for pushing gel with five runs executed at each pushing force. For pushing forces below 13 nN, the motion is erratic in direction and magnitude, so no data was taken. For pushing forces above 72 nN, the motion is too fast to reliably push a microgel without flipping it on its edge. Results show that the pushing speed of a microgel (gel style F in Supplementary Table 1 ) by a micro-robot increased linearly with the magnetic force exerted ( Fig. 1e ). We also observed that the manipulation speed is not greatly affected by hydrogel shape or size, and that there is no significant variation in pushing speed for a single type of a gel ( Supplementary Fig. 1 ). Figure 1: Fabrication and micro-robotic coding of cell-encapsulating hydrogels. ( a ) Cell-encapsulating hydrogel fabrication via ultraviolet (UV) photocrosslinking. ( b ) Fabricated hydrogels and micrograph of L-shaped hydrogels. Scale bar, 1 mm. ( c ) Magnetic coil system used to drive magnetic micro-robots remotely. All system components are shown with the coils in the operational position. Two coils hinge open to allow for access to the workspace. ( d ) Motion of untethered magnetic micro-robot and coding of building units, for example soft hydrogels or rigid micro-components. Scale bar, 1 mm. ( e ) The pushing speed of a microgel (gel style F in Supplementary Table 1 ) by a 750 μm × 750 μm × 225 μm micro-robot moving on a planar glass surface in phosphate-buffered saline solution. Error bars represent standard error of the mean. The micro-robot motion was guided by a magnetic force of varying magnitude. Average speed is shown for pushing gel with five runs executed at each pushing force. For pushing forces below 13 nN, the motion is erratic in direction and magnitude, so no data was taken. For pushing forces above 72 nN, the motion is too fast to reliably push a microgel without flipping it on its edge. Full size image 2D micro-robotic coding of material composition We precisely coded Poly(ethylene glycol) dimethacrylate (PEG) hydrogels on-demand into different geometrical shapes using the magnetic micro-robot ( Fig. 2 ). Images of hydrogels coded into a variety of final geometries such as plus, square and rod shapes are shown in Fig. 2a–f . The robotic manipulation approach is capable of dynamically reconfiguring the material morphology ( Supplementary Movie 1 ). As such, Fig. 2a–f represents a continuous sequence, where one shape is built (for example, square in Fig. 2c ) and then reconfigured into the next shape (for example, plus shape in Fig. 2d ). This capability could be critical for cellomics, system biology studies and microphysiological system engineering applications [20] where a temporal component is beneficial (for example, introducing building blocks that encapsulates certain types of cells with biomolecules, such as inhibitors, growth factors and drugs). To illustrate the capability of the micro-robot in handling hydrogel units of different shapes and weights in one coding sequence, we patterned triangular, square, plus-shaped, bracket-shaped ( Supplementary Movie 2 ) and circular PEG hydrogels into composite forms with interconnected micro-components ( Fig. 2g–j ). To further demonstrate the scalability of the technology, we coded gels into configurations of a variety of shapes, made from more than 20 building units ( Fig. 2k ). Similar manipulation was performed for gels of diverse shapes made from gelatin methacrylate (GelMA) ( Fig. 2l–t ). To demonstrate the dynamic orientation control capability of untethered micro-robots for manipulating and coding a variety of microscale objects made of different materials and by different fabrication processes, we fabricated a 20 mm × 20 mm × 4 mm reservoir and ‘tetris’-shaped PEG hydrogel units ( Supplementary Movie 3 ). Snapshots of manipulation and coding of these PEG hydrogels in a rectangular reservoir at different time points are shown ( Fig. 2u–y ). This task required the orientation and position of each incoming building unit to be adjusted dynamically by the micro-robot, as the geometry of available cavities changed dynamically after each operation. 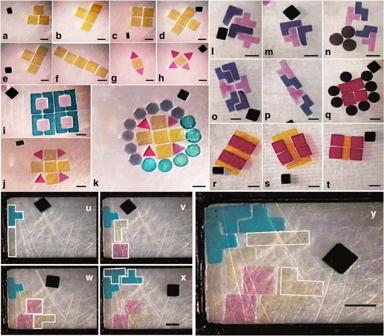Figure 2: Two-dimensional micro-robotic coding of material composition. Micro-robotic coding and reconfiguration of Poly(ethylene glycol) dimethacrylate hydrogels (a–k) and gelatin methacrylate hydrogels (l–t) with various shapes into complex planar constructs. The black object in each image is top-view of a crawling micro-robot. To demonstrate the precision of micro-robotic manipulation, gels with several shapes including square, triangle, circle, hexagon, bracket-shape, plus-shape and others were coded. All the experiments were performed in 20 mm × 20 mm × 4 mm chamber in phosphate-buffered saline (PBS). Continuous coding and reconfiguring sequences are shown in panes (a–f), (g,h), (j,k), (l–p) and (r–t). Orientation and position control in untethered micro-robotic coding of material composition (u–y). Snapshots of ‘tetris’-shaped PEG hydrogels in a rectangular reservoir at different time points: 2:08 (u), 8:32 (v), 16:12 (w), 31:39 (x), 48:00 (y) in minutes:seconds format. Orientation and position of incoming hydrogels were dynamically changed as the geometry of cavities dynamically changed. All the experiments were performed in a 20 mm × 20 mm × 4 mm chamber. Scale bar, 1 mm. Figure 2: Two-dimensional micro-robotic coding of material composition. Micro-robotic coding and reconfiguration of Poly(ethylene glycol) dimethacrylate hydrogels ( a – k ) and gelatin methacrylate hydrogels ( l – t ) with various shapes into complex planar constructs. The black object in each image is top-view of a crawling micro-robot. To demonstrate the precision of micro-robotic manipulation, gels with several shapes including square, triangle, circle, hexagon, bracket-shape, plus-shape and others were coded. All the experiments were performed in 20 mm × 20 mm × 4 mm chamber in phosphate-buffered saline (PBS). Continuous coding and reconfiguring sequences are shown in panes ( a – f ), ( g , h ), ( j , k ), ( l – p ) and ( r – t ). Orientation and position control in untethered micro-robotic coding of material composition ( u – y ). Snapshots of ‘tetris’-shaped PEG hydrogels in a rectangular reservoir at different time points: 2:08 ( u ), 8:32 ( v ), 16:12 ( w ), 31:39 ( x ), 48:00 ( y ) in minutes:seconds format. Orientation and position of incoming hydrogels were dynamically changed as the geometry of cavities dynamically changed. All the experiments were performed in a 20 mm × 20 mm × 4 mm chamber. Scale bar, 1 mm. Full size image Versatility of micro-robotic coding Untethered micro-robotic coding can also be applied to rigid micro-objects made from a variety of materials. We demonstrated the coding of silicon chiplets (see Methods for details) and PDMS blocks ( Supplementary Fig. 2 ; see Methods for details) into square, triangle and rod patterns in Fig. 3 , which shows snapshots of these 2D manipulation and coding processes. These results show that the presented micro-robotic coding technology holds great potential for broader applications in the coding and repair of microscale components. 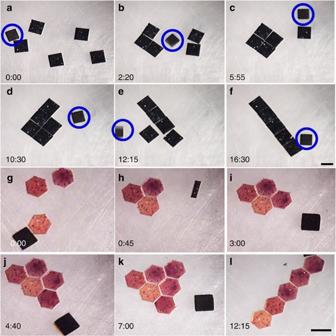Figure 3: Versatility of micro-robotic coding. Micro-robotic coding of (a–f) square silicon chiplets into square and rod patterns, and (g–l) hexagonal polydimethylsiloxane blocks into triangle and rod patterns. All the experiments were performed in a 20 mm × 20 mm × 4 mm chamber. Snapshots of manipulation of 1 mm × 1 mm square silicon chiplets at different time points (shown at the left corner). The time stamp format is minutes:seconds. The magnetic micro-robots are shown in a blue circle (a–f). Black object in each image (g–l) is top-view of the crawling magnetic micro-robot. Scale bar, 1 mm. Figure 3: Versatility of micro-robotic coding. Micro-robotic coding of ( a – f ) square silicon chiplets into square and rod patterns, and ( g – l ) hexagonal polydimethylsiloxane blocks into triangle and rod patterns. All the experiments were performed in a 20 mm × 20 mm × 4 mm chamber. Snapshots of manipulation of 1 mm × 1 mm square silicon chiplets at different time points (shown at the left corner). The time stamp format is minutes:seconds. The magnetic micro-robots are shown in a blue circle ( a – f ). Black object in each image ( g – l ) is top-view of the crawling magnetic micro-robot. Scale bar, 1 mm. Full size image 3D micro-robotic coding of material composition The micro-robotic manipulation approach can also be extended to 3D coding. Here, layered 3D complex materials were created in a confined area using raised plateaus and ramps ( Supplementary Movie 4 ). This strategy allowed the micro-robot to simply push gels to a desired height, where they can be placed onto an existing gel layer. The results, shown in Fig. 4a–g , demonstrate three layers of hydrogels built into a pyramid shape. In Fig. 4e,f , the upper two layers were moved to a new location as a demonstration of the reconfigurable nature of the robotic coding method. A schematic illustration of the coded pyramid is shown in Fig. 4g . In Fig. 4h–l , a heterogeneous structure was created with hydrogels encapsulating copper rods of diameter 10 μm and polystyrene spheres of diameter 200 μm. These objects were encased by gels on either side and on top to create complex repeating 3D morphologies using the versatility of an untethered micro-robot agent. Within a continuous process, the micro-robot is able to incorporate 3D objects of various sizes and shapes into one structure. 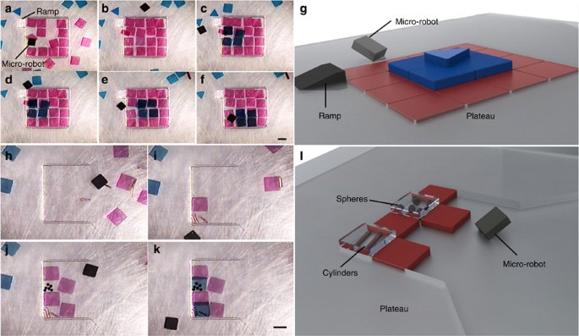Figure 4: Three-dimensional micro-robotic coding of material composition. Micro-robotic creation of (a–g) a three-layer heterogeneous pyramid structure consisting of 16, 4 and 1 gel on each layer, and (h–l) a heterogeneous structure consisting of poly(ethylene glycol) dimethacrylate (PEG) hydrogels, which totally encase 100 μm diameter copper cylinders and 200 μm diameter polystyrene spheres. All the experiments were performed in a 20 mm × 20 mm × 4 mm chamber in phosphate-buffered saline (PBS). Snapshots of manipulation stages are shown in each subfigure, with the completed structure shown in schematic form in (g) and (l), corresponding to panes (e) and (k), respectively. Gels were placed on the second layer by moving them over a polyester plateau, which is the same thickness as the first layer of gels. The third layer was reached in (d) by pushing the gels up a polyester ramp. The time points of images are: 2:45 (a), 12:48 (b), 19:24 (c), 21:19 (d), 22:28 (e), 25:22 (f), 0:00 (h), 3:40 (i), 13:36 (j) and 15:39 (k) in minutes:seconds format. Scale bar, 1 mm. Figure 4: Three-dimensional micro-robotic coding of material composition. Micro-robotic creation of ( a – g ) a three-layer heterogeneous pyramid structure consisting of 16, 4 and 1 gel on each layer, and ( h – l ) a heterogeneous structure consisting of poly(ethylene glycol) dimethacrylate (PEG) hydrogels, which totally encase 100 μm diameter copper cylinders and 200 μm diameter polystyrene spheres. All the experiments were performed in a 20 mm × 20 mm × 4 mm chamber in phosphate-buffered saline (PBS). Snapshots of manipulation stages are shown in each subfigure, with the completed structure shown in schematic form in ( g ) and ( l ), corresponding to panes ( e ) and ( k ), respectively. Gels were placed on the second layer by moving them over a polyester plateau, which is the same thickness as the first layer of gels. The third layer was reached in ( d ) by pushing the gels up a polyester ramp. The time points of images are: 2:45 ( a ), 12:48 ( b ), 19:24 ( c ), 21:19 ( d ), 22:28 ( e ), 25:22 ( f ), 0:00 ( h ), 3:40 ( i ), 13:36 ( j ) and 15:39 ( k ) in minutes:seconds format. Scale bar, 1 mm. Full size image Spatially coded constructs for tissue culture The patterning of cell-encapsulating hydrogels is an important task with broad applications in regenerative medicine, cell-based pharmaceutical research and tissue engineering [9] . Application of our untethered micro-robotic coding approach offers a high level of control over complex tissue architectures. 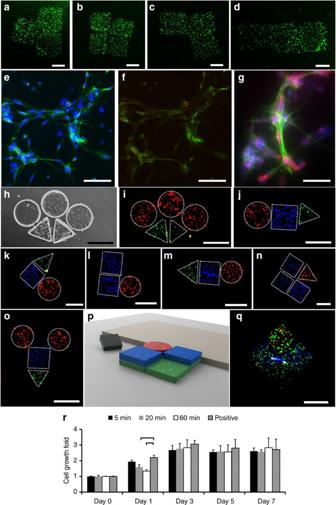Figure 5: Spatially coded constructs for tissue culture. Fluorescence images of National Institutes of Health (NIH) 3T3 mouse embryonic fibroblast cell-encapsulating hydrogels after the assembly of (a) T-shape, (b) square-shape, (c) L-shape and (d) rod-shape constructs. Scale bar, 500 μm for (a–d). Green represents live cells and red represents dead cells. (e–g) Immunocytochemistry of proliferating cells stained with Ki67 (red), DAPI (blue) and Phalloidin (green) at day 4. (e) Cells stained with DAPI and Phalloidin at × 20 magnification. Scale bar, 100 μm. (f) Cells stained with Ki67 and Phalloidin at × 20 magnification. Scale bar, 100 μm. (g) Cells stained with Ki67, DAPI and Phalloidin at × 40 magnification. Scale bar, 40 μm. (a–g) Stainings were performed following the assembly of hydrogels. (h–q) Two- and three-dimensional heterogeneous assemblies of human umbilical vein endothelial cells, 3T3 and cardiomyocyte-encapsulating hydrogels. HUVECs, 3T3s and cardiomyocytes are stained with Alexa 488 (green), DAPI (blue) and propidium iodide (red), respectively. (h) Bright field and (i) fluorescence images of an assembly composed of circular and triangular gels. (j–o) Fluorescence images of several two-dimensional heterogeneous assemblies of HUVEC, 3T3 and cardiomyocyte-encapsulating hydrogels. (p) Schematic form and (q) fluorescence image of three-dimensional heterogeneous assembly of HUVEC, 3T3 and cardiomyocyte encapsulating hydrogels. Scale bar, 500 μm for (h–q). Stainings were performed before the assembly of hydrogels for (h–q). Teleoperated assembly durations of (a–d,h–q) are ~10 s to 5 min depending on the complexity of the final shape. (r) MTT (3-(4,5-dimethylthiazol-2-yl)-2,5-diphenyltetrazolium bromide, a yellow tetrazole) assay results of 3T3 cell suspensions in which micro-robots were kept for 5, 20 and 60 min durations. The positive control represents the cells that were incubated without any micro-robot presence. Results are normalized with day 0 absorbance values. Statistical analysis was only performed between positive control and (5, 20, 60) min cases. Brackets connecting groups indicate statistically significant difference (n=6,P<0.05). Error bars represent standard error of the mean. Figure 5 shows the results of cell viability and proliferation using fluorescence imaging after robotic manipulation. Cell viability is quantified in Fig. 5a–d for assemblies of three and four hydrogels containing NIH 3T3 cells. Immunocytochemistry results for groups of two and three assembled gels are shown in Fig. 5e–g , demonstrating the proliferation of cells within the gels on day 4 after robotic coding. Cells were stained with Ki67 (red), DAPI (blue) and Phalloidin (green) in Fig. 5e–g . To show the heterogeneous coding capability of the approach, we performed 2D and 3D assembly of human umbilical vein endothelial cells (HUVECs), 3T3 fibroblasts and cardiomyocyte-encapsulating hydrogels ( Fig. 5h–q ). HUVEC, 3T3 and cardiomyocyte cells were stained with Alexa 488 (green), DAPI (blue) and propidium iodide (red), respectively. Further, the cytocompatibility of the micro-robot is studied in Fig. 5r , where MTT assay results were taken for cell suspensions that were directly exposed to a micro-robot for 5, 20 and 60 min (see MTT assays section). Results show that cells proliferated over days (up to 7 days), and there is only statistically significant difference at day 1 among the control and other groups. These results demonstrate that the micro-robotic coding method is viable for biological constructs and can be used without causing long-term effects to the biological growth. Figure 5: Spatially coded constructs for tissue culture. Fluorescence images of National Institutes of Health (NIH) 3T3 mouse embryonic fibroblast cell-encapsulating hydrogels after the assembly of ( a ) T-shape, ( b ) square-shape, ( c ) L-shape and ( d ) rod-shape constructs. Scale bar, 500 μm for ( a – d ). Green represents live cells and red represents dead cells. ( e – g ) Immunocytochemistry of proliferating cells stained with Ki67 (red), DAPI (blue) and Phalloidin (green) at day 4. ( e ) Cells stained with DAPI and Phalloidin at × 20 magnification. Scale bar, 100 μm. ( f ) Cells stained with Ki67 and Phalloidin at × 20 magnification. Scale bar, 100 μm. ( g ) Cells stained with Ki67, DAPI and Phalloidin at × 40 magnification. Scale bar, 40 μm. ( a – g ) Stainings were performed following the assembly of hydrogels. ( h – q ) Two- and three-dimensional heterogeneous assemblies of human umbilical vein endothelial cells, 3T3 and cardiomyocyte-encapsulating hydrogels. HUVECs, 3T3s and cardiomyocytes are stained with Alexa 488 (green), DAPI (blue) and propidium iodide (red), respectively. ( h ) Bright field and ( i ) fluorescence images of an assembly composed of circular and triangular gels. ( j – o ) Fluorescence images of several two-dimensional heterogeneous assemblies of HUVEC, 3T3 and cardiomyocyte-encapsulating hydrogels. ( p ) Schematic form and ( q ) fluorescence image of three-dimensional heterogeneous assembly of HUVEC, 3T3 and cardiomyocyte encapsulating hydrogels. Scale bar, 500 μm for ( h – q ). Stainings were performed before the assembly of hydrogels for ( h – q ). Teleoperated assembly durations of ( a – d , h – q ) are ~10 s to 5 min depending on the complexity of the final shape. ( r ) MTT (3-(4,5-dimethylthiazol-2-yl)-2,5-diphenyltetrazolium bromide, a yellow tetrazole) assay results of 3T3 cell suspensions in which micro-robots were kept for 5, 20 and 60 min durations. The positive control represents the cells that were incubated without any micro-robot presence. Results are normalized with day 0 absorbance values. Statistical analysis was only performed between positive control and (5, 20, 60) min cases. Brackets connecting groups indicate statistically significant difference ( n =6, P <0.05). Error bars represent standard error of the mean. Full size image The current throughput of the teleoperated 3D micro-robotic assembly is limited by the use of a single robot. Such throughput is suitable as a scientific tool for the study of spatiotemporal effects of bioactive molecules, or microenvironmental changes on tissue growth or cellular processes [21] . For applications that require assembly operations of a larger volume, the assembly throughput could be improved by assembly automation and parallel actuation using a large number of micro-robots working as a team. In this direction, viable methods are reported to both automate assembly of micro-parts using visual feedback [22] and control a team of magnetic micro-robots for addressable actuation towards parallel assembly [23] , [24] , [25] . In comparison with pick-and-place manipulation methods, the presented contact-based micromanipulation approach cannot grasp or lift the micro-components. However, with the correct system of ramps and plateaus, it is expected that a 3D assembly of up to five layers could be achieved using the presented method. The process to build multiple layers is limited by the support of lower gel layers and the ability of the micro-robot to push gels up to higher layers. Blocks that encapsulate different cell lines can be coded onto microchips by the presented method to bioengineer microphysiological systems with broad applications. For instance, spatiotemporal manipulation of the microenvironment can be used to investigate numerous biological processes such as the effect of growth factors on various cell types. Such applications can be investigated by positioning growth-factor-encapsulating hydrogels in the vicinity of other cell-encapsulating hydrogels. The growth-factor-loaded gels can then be removed or repositioned to investigate spatiotemporal effects. In a previous study [8] , it was shown that placing a relatively large microgel next to a small one encapsulating a neuron resulted in selective axonal growth towards the larger gel. The presented robotic approach here can potentially perform dynamical changes in such neural microenvironments, which are not possible by photolithography or bioprinting. Therefore, the new capabilities allowing reconfigurability and reversibility of microcomponent placement can broadly enable researchers to study several transient biological problems in addition to bottom-up tissue engineering. In summary, we have presented an untethered micro-robotic approach that provides temporal and spatial control to code micro- or millimeter-scale building blocks such as rigid copper bars, polystyrene beads, silicon chiplets and cell-encapsulating hydrogels into reconfigurable heterogeneous materials in 2D and 3D. We demonstrated that the manipulation method can be used with cell-encapsulating microgels without affecting cell viability and proliferation. Magnetic micro-robots could provide additional functionality as in situ tools, for example, by functionalizing with on-board cell-encapsulating hydrogels for toxicity detection. In addition, the coding and manipulation methodology developed here can find broad applications in areas such as regenerative medicine, microphysiological system engineering, pharmaceutical research, biological research and microscale manufacturing. Fabrication of microgels PEG precursor solution was prepared by dissolving (20%, wt/wt) Poly(ethylene glycol) dimethacrylate (PEGDMA; MW 1,000; Polysciences) in Dulbecco’s phosphate-buffered saline (DPBS, GIBCO). GelMA precursor solution was prepared by dissolving (5%, wt/wt) GelMA foam-like powder in DPBS (GIBCO). Then, 2-hydroxy-1-(4-(hydroxyethoxy)phenyl)-2-methyl-1-propanone photoinitiator (1%, wt/wt, Irgacure 2959; CIBA Chemicals) was added to the prepolymer solution. In this study, we used photomasks with several geometries ( Fig. 2 ). A 50 μl droplet of photocrosslinkable prepolymer solution was pipetted onto a glass slide covered by a cover slip and separated by spacers (cover slip 25 × 25 mm 2 , thickness: 150 μm). The photomasks were placed on the cover slip between the UV light and prepolymer. Another 25 × 25 mm 2 coverslide was placed onto the droplet. Microgels were fabricated by exposing the gel prepolymer solution to UV light (500 mW; at a height of 50 mm above the microgels) for 30 s, for polymerization to take place on the surface of the glass slide. Then, the photomask and glass cover slip were removed. Using a scalpel, the microgels were removed and left to soak in DPBS solution in a standard 60 mm Petri dish (Fisher Scientific). Fabrication of silicon chiplets Silicon chiplets (1 mm × 1 mm × 0.1 mm) were fabricated from 2-inch silicon wafers (University Wafer, MA) by automatic dicing saw (Model DAD321, Disco Corp., Tokyo, Japan). Fabrication of PDMS building blocks PDMS building blocks were fabricated using photolithography and rapid prototyping with minor modifications [26] ( Supplementary Fig. 2 ). Briefly, an SU-8 master mould with a thickness of 500 μm was fabricated on a 4-inch silicon wafer using standard photolithography. Before use, the master mould was coated with a layer of Trichloro(1H,1H,2H,2H-perfluorooctyl)silane (Sigma) to ease the release of the PDMS structure. PDMS prepolymer was prepared by mixing PDMS precursor and curing agent in a ratio of 11:1. The PDMS mould was fabricated by curing the prepolymer on the master mould at 80 °C for 1 h. Before use, the PDMS mould was coated with a layer of Trichloro(1H,1H,2H,2H-perfluorooctyl)silane to ease the release of the PDMS blocks. PDMS prepolymer for the building blocks was prepared by mixing PDMS precursor and curing agent in a ratio of 9:1. Sudan Red G (Sigma) was mixed with the prepolymer with a final concentration of 0.5% (w/w) for visualization of the PDMS blocks. The prepolymer was poured on the PDMS mould, followed by removal of the excess prepolymer using a razor blade. The prepolymer was cured at 80 °C for 1 h in an oven. The final PDMS blocks were released by bending the PDMS mould. PDMS blocks were made hydrophilic by oxygen plasma treatment before coding experiments. Experimental setup The fabricated building blocks (for example, microgels, silicon chiplets, PDMS blocks) were suspended in DPBS solution in petri dishes. They were coded into various complex shapes with a system of eight electromagnets ( Fig. 1c ). Building units were directed towards a prespecified location one-by-one through direct pushing by a magnetic untethered micro-robot. Magnetic micro-robots are actuated by a set of independent electromagnetic coils, aligned pointing towards a common center point, with an open space of ~10.4 cm. The coils are operated with an air or iron core, depending on the desired magnetic fields and gradients. The maximum fields produced by the system driven at maximum current (19 A each) are 8.3 mT using air cores and 24.4 mT using iron cores. Similarly, maximum field spatial gradients are 0.34 T m −1 using air cores and 1.02 T m −1 using iron cores. Fields and field gradients are linearly related to the coil currents, and are measured using a Hall effect sensor (Allegro A1321) with an error of about 0.1 mT. Control of the currents driving the electromagnetic coils is performed by a PC with data acquisition system at a control bandwidth of 20 kHz, and the coils are powered by linear electronic amplifiers (SyRen 25). Magnetic micro-robots can be controlled by the magnetic coils surrounding the workspace. The total magnetic torque T and force F that govern these interactions are: for a micro-robot with magnetization M , where B is the total magnetic field from the coils. Micro-robot actuation is performed by a combination of magnetic forces that directly pull in the plane of the substrate, and magnetic torques that act to break the surface friction and adhesion with the surface. These torques are applied as a sawtooth wave at a frequency of 10–50 Hz and result in discrete micro-robot steps of about 10–300 μm depending on pulse magnitude and frequency. Fabrication of magnetic micro-robots In this work, individual micro-robots were fabricated to be magnetically hard, retaining their internal magnetization in the absence of an externally applied magnetic field. Micro-robots were fabricated in a batch process using soft photolithography and moulding techniques [27] . Micro-robots were composed of NdFeB particles in a polyurethane (BJB Enterprise, ST-1087) matrix, with fabrication details given in ref. 28 . In short, soft rubber moulds were made from replica moulding of SU-8 features patterned using photolithography on a silicon substrate ( Supplementary Fig. 2 ). Micro-robots were created from the mould by pouring the NdFeB–polyurethane slurry into the mould. Owing to the high magnetic coercivity of NdFeB (that is, fields over 600 mT are required to demagnetize NdFeB), these micro-robots were not subject to demagnetization from the relatively weak fields applied in this work. Nominal micro-robot volume magnetization M was about 50 kA m −1 as measured in an alternating gradient force magnetometer (Princeton Measurements MicroMag 2900). The moulding process for all micro-robots was prone to variations in micro-robot geometry (up to about 10% from nominal), but the motion control method was not sensitive to small geometric changes. Secondary crosslinking to stabilize the coded construct The microgels were coded on the bottom surface of the reservoir and 10 μl prepolymer solution was added to the final construct. The microgels were exposed to secondary UV crosslinking for 20 s to stabilize the shape of the structure. Cell encapsulation NIH 3T3 fibroblasts were cultured in Dulbecco’s modified Eagle’s medium (DMEM; Sigma-Aldrich) supplemented with 10% fetal bovine serum (FBS; GIBCO) in a 5% CO 2 -humidified incubator at 37 °C. To collect and encapsulate cells, the cells were first trypsinized with 1% trypsin (GIBCO) and centrifuged at 1,000 r.p.m. for 5 min. The cells were suspended in 5% w/v GelMA dissolved in PBS (Gibco, Invitrogen) at a density of 1 × 10 7 per ml, and mixed with 0.5% w/v of photoinitiator (Irgacure, Ciba). Cell-encapsulating microgels were then fabricated via photocrosslinking with 500 mW UV light for 20 s ( Fig. 1a ). The cell-encapsulating microgels were first washed with DPBS and then incubated with live/dead dyes for 15 min. The live/dead dyes were prepared by diluting 2 ml of calcein AM, and 0.5 ml of ethidium homodimer-1 (Molecular Probes) in 1 ml of DPBS. Cells were labelled green with Calcein AM and labelled red with PKH26 red fluorescent cell linker. The fluorescent images were taken using an inverted fluorescent microscope (Nikon, TE2000). Immunocytochemistry images were taken after 4 days of culture at 37 °C, 5% CO 2 in humidified incubator. Staining hydrogels To increase visibility during video recording, hydrogels were stained with food dye (Procion Mx dye), which is composed of small molecules and has a minor interaction with the polymer. The dye demonstrated enough interaction to stay for a sufficiently long time in the hydrogel for the coding process and can be seen during the video recording. Image recording and processing The videos were recorded by a digital camera (Foculus F0134SB) connected to variable magnification microscope lenses, providing up to a 26 mm × 20 mm field of view from the top perspective. Cell viability was quantified by analysing the images using public domain NIH ImageJ program (developed at the U.S. National Institutes of Health and available at http://rsb.info.nih.gov/nih/image/ ). To calculate micro-robot velocity from video, a tracking algorithm based on a particle filter was used. This algorithm finds the most likely micro-robot position, and filters the position using a low-pass butterworth filter to reduce tracking noise. Immunocytochemistry staining for UV crosslinked gels Proliferating cells encapsulated into hydrogels were detected with Ki67 immunocytochemistry. Assembled 3T3 cell-encapsulating gels ( Fig. 5a–g ) were fixed with 1% paraformaldehyde for 1 h at room temperature and washed. Gels were permeabilized with 0.3% Triton X-100 (Sigma), in 1% BSA (Sigma), for minimum 1 h at room temperature. Gels were stained with Ki67 (Ab16667, Abcam) overnight at 4 °C. After washing, gels were incubated with secondary antibody goat anti rabbit Alexa Fluor 564 (A11011, Invitrogen) for 2 h at room temperature. Actin cytoskeleton was stained with Phalloidin Alexa Fluor 488 (Invitrogen), and DAPI was used as nuclear counter staining. After washing, hydrogels were visualized under fluorescent microscope (Zeiss AXIO). Fluorescence staining for heterogeneous assemblies HUVEC, 3T3 fibroblast and chicken cardiomyocyte-encapsulating hydrogels were fixed with 1% paraformaldehyde for 1 h at room temperature and washed. Gels were permeabilized with 0.3% Triton X-100 (Sigma), in 1% BSA (Sigma) blocking solution, for minimum 1 h at room temperature. Cardiomyocytes were stained with ethidium homodimer-1 (Life Technologies). HUVECs were stained with Alexa Fluor 488 Phalloidin (Life Technologies). 3T3 fibroblasts were stained with DAPI (Life Technologies). After washing, hydrogels were imaged with fluorescent microscope (Zeiss AXIO). The stained cell-encapsulating gels were then assembled by the micro-robot with precision ( Fig. 5h–q ). MTT assays NIH 3T3 cells were cultured in Dulbecco’s modified Eagle’s medium (DMEM) supplemented with 10% fetal bovine serum and 1% penicillin–streptomycin mixture in a humidified and 5% CO 2 -containing atmosphere at 37 °C. For MTT viability assay, cells were seeded in a 96-well plate with the density of 10 5 cells ml −1 (in a total volume of 100 μl cell suspension per well). When the cells were attached after 4 h, one micro-robot was placed into each well. The cells were incubated for 5, 20 and 60 min at 37 °C. After incubations, micro-robots were removed and cell culture medium was aspirated from the wells for all samples. Then, fresh cell culture medium and MTT reagent (10% v/v) were added and incubated for 4 h. At the end of 4 h the resulting formazan was dissolved in 100 μl MTT-solubilizing reagent SDS. Absorbance of the induced formazan dye was measured by BMG FLUOstar Galaxy-Multi-functional Microplate Reader on the next day. All determinations were carried out in six repeats for each sample and three independent experiments were carried out. MTT proliferation assays were performed 0, 1, 3, 5 and 7 days after the removal of micro-robots from cell suspensions. Cells without any micro-robot presence were used as control. Statistical methods Fluorescent intensity measurements obtained from MTT assay ( n =12–15) were statistically compared using parametric one way analysis of variance (ANOVA) with Tukey’s posthoc test for multiple comparisons. Statistical significance threshold was set at 0.05 ( P <0.05). How to cite this article: Tasoglu, S. et al . Untethered micro-robotic coding of three-dimensional material composition. Nat. Commun. 5:3124 doi: 10.1038/ncomms4124 (2014).